Regulation of histone modification and chromatin structure by the p53–PADI4 pathway Histone proteins are modified in response to various external signals; however, their mechanisms are still not fully understood. Citrullination is a post-transcriptional modification that converts arginine in proteins into citrulline. Here we show in vivo and in vitro citrullination of the arginine 3 residue of histone H4 (cit-H4R3) in response to DNA damage through the p53–PADI4 pathway. We also show DNA damage-induced citrullination of Lamin C. Cit-H4R3 and citrullinated Lamin C localize around fragmented nuclei in apoptotic cells. Ectopic expression of PADI4 leads to chromatin decondensation and promotes DNA cleavage, whereas Padi4 −/− mice exhibit resistance to radiation-induced apoptosis in the thymus. Furthermore, the level of cit-H4R3 is negatively correlated with p53 protein expression and with tumour size in non-small cell lung cancer tissues. Our findings reveal that cit-H4R3 may be an 'apoptotic histone code' to detect damaged cells and induce nuclear fragmentation, which has a crucial role in carcinogenesis. In response to DNA damage, various protein kinases phosphorylate p53 at its amino terminus leading to the stabilization and accumulation of p53 protein [1] , [2] . As a guardian of the genome, p53 transactivates a number of its target genes to induce cell-cycle arrest or apoptosis and subsequently eliminates cells with risk of malignant transformation [3] . Morphological changes such as chromatin condensation, DNA laddering, nuclear lamina breakdown and nuclear fragmentation are characteristic of apoptotic cell death, although the role of p53 during these dynamic nuclear events has not been elucidated. We have isolated a number of p53-target genes including p53AIP1, p53R2, p53RDL1 and XEDAR [4] , [5] , [6] , [7] , [8] , [9] , and implicated the molecular mechanisms by which p53 regulated the cell fate, death or survival, by regulating the expression levels of these genes. We recently reported a p53-regulated posttranscriptional modification of many proteins through the transcriptional regulation of PADI4 (ref. 10 ) that converts an arginine residue in proteins to a citrulline residue, known as citrullination or deimination [11] . This reaction is mediated by the Ca 2+ -dependent enzyme peptidylarginine deiminase. Citrullination of proteins causes a loss of positive charge and results in a significant biochemical effect. Bacterial infection has been indicated to stimulate PADI4-mediated hypercitrullination of histones in neutrophils and subsequently promoted highly decondensed extracellular chromatin structure called NET (neutrophil extracellular trap) that could capture and kill microorganisms [12] , [13] . On the other hand, citrullinated peptides/proteins are recognized as non-self proteins and subsequently activate immune systems. Citrullinated myelin basic protein in the brain is considered as a putative autoantigen associated with multiple sclerosis [14] . In addition, autoantibodies against citrullinated peptides derived from filaggrin or fibrin have been established as specific markers for rheumatoid arthritis [15] , [16] , [17] . Furthermore, we have revealed that a functional haplotype of the PADI4 gene is associated with rheumatoid arthritis [18] . Thus, activated PADI4 function has been shown to be associated with the pathogenesis of rheumatoid arthritis through induction of the antigenicity of proteins. Here we investigate the physiological role of p53–PADI4 signalling in the DNA damage response by using PADI4 deficient mice as well as clinical cancer tissues. In this study, we revealed the crucial role of PADI4 in the apoptotic pathway and human carcinogenesis. Citrullination of core histones in response to DNA damage As histones H3 and H4 were shown to be citrullinated by PADI4 (refs 19 , 20 ), we assessed whether core histones are citrullinated in response to DNA damage. Acid-extracted histones from adriamycin (ADR)-treated U-2 OS cells were immunoblotted with an antibody against a chemically modified form of citrulline (anti-MC antibody). Western blot analysis revealed the citrullination of three of four core histones in a PADI4-dependent manner ( Fig. 1a,b ). Ectopic expression of PADI4 also induced the citrullination of at least two core histones ( Fig. 1c ). To further characterize this modification, purified histones were treated with recombinant PADI4. Antibodies against specific citrulline residues (cit-H3R2,8,17 or cit-H4R3) as well as anti-MC antibody could detect PADI4-treated histones H3 and H4, respectively ( Fig. 1d ). Interestingly, anti-cit-H4R3 antibody cross-reacted with citrullinated H2A, probably owing to the high similarity between histones H4 and H2A ( Fig. 1d,e ). 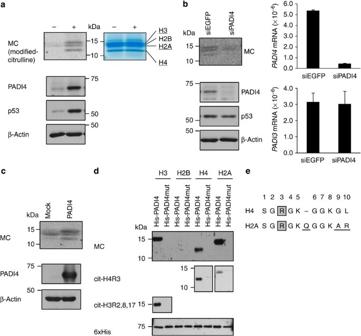Figure 1: Citrullination of core histones in the damaged cells. (a) Histones extracted from U-2 OS cells 48 h after ADR treatment (lane 2) were immunoblotted with anti-modified citrulline (anti-MC) antibody (left panel). U-2 OS cells without ADR treatment were used as a negative control (lane 1). CBB stain is shown in the right panel to ensure equal loading. Whole-cell extracts were subjected to immunoblotting with anti-PADI4, anti-p53 or anti-β-actin antibody. (b) siRNA against PADI4 was trasfected 10 h before DNA damage treatment. siEGFP was used as a control. Purified histones were immunoblotted with anti-MC antibody (upper left panel). Whole-cell extracts were subjected to immunoblotting with anti-PADI4, anti-p53 or anti-β-actin antibody (lower left panel). Quantitative PCR analysis ofPADI4orPADI3expression (right panel). Error bars represent range (n=2).GAPDHwas used for normalization of expression levels. (c) Histones were extracted from PADI4-introduced or mock-transfected HEK293T cells, and immunoblotted with anti-MC antibody. Whole-cell extracts were subjected to immunoblotting with anti-PADI4 or anti-β-actin antibody. (d)In vitrocitrullination followed by western blotting with anti-MC, anti-citrullinated histone H4R3 (cit-H4R3), anti-citrullinated histone H3R2,8,17 (cit-H3R2,8,17), or anti-His-tag (6×His) antibody. Each recombinant histone was incubated with wild-type or mutant PADI4 protein in the presence of 10−3M of calcium at 37 °C for 1 h. (e) Alignment of amino-acid sequences of the N-terminal regions of histone H2A and H4. Figure 1: Citrullination of core histones in the damaged cells. ( a ) Histones extracted from U-2 OS cells 48 h after ADR treatment (lane 2) were immunoblotted with anti-modified citrulline (anti-MC) antibody (left panel). U-2 OS cells without ADR treatment were used as a negative control (lane 1). CBB stain is shown in the right panel to ensure equal loading. Whole-cell extracts were subjected to immunoblotting with anti-PADI4, anti-p53 or anti-β-actin antibody. ( b ) siRNA against PADI4 was trasfected 10 h before DNA damage treatment. siEGFP was used as a control. Purified histones were immunoblotted with anti-MC antibody (upper left panel). Whole-cell extracts were subjected to immunoblotting with anti-PADI4, anti-p53 or anti-β-actin antibody (lower left panel). Quantitative PCR analysis of PADI4 or PADI3 expression (right panel). Error bars represent range ( n =2). GAPDH was used for normalization of expression levels. ( c ) Histones were extracted from PADI4-introduced or mock-transfected HEK293T cells, and immunoblotted with anti-MC antibody. Whole-cell extracts were subjected to immunoblotting with anti-PADI4 or anti-β-actin antibody. ( d ) In vitro citrullination followed by western blotting with anti-MC, anti-citrullinated histone H4R3 (cit-H4R3), anti-citrullinated histone H3R2,8,17 (cit-H3R2,8,17), or anti-His-tag (6×His) antibody. Each recombinant histone was incubated with wild-type or mutant PADI4 protein in the presence of 10 −3 M of calcium at 37 °C for 1 h. ( e ) Alignment of amino-acid sequences of the N-terminal regions of histone H2A and H4. Full size image p53–PADI4 citrullinates histone H4R3 Western blotting of core histone proteins purified from ADR-treated U-2 OS cells indicated citrullination of H4R3 by DNA damage ( Fig. 2a ), but the citrullination was blocked by small interfering RNA (siRNA) against p53 or PADI4 ( Fig. 2b ). Concordantly, ectopic introduction of PADI4 into cells induced the citrullination of H4R3 ( Fig. 2c ). Although PADI4 was reported to function as demethylase of mono-methyl-H4R3 in vitro [19] , [20] , PADI4 activation did not affect H4R3 methylation status in our experimental system ( Supplementary Fig. S1 ). 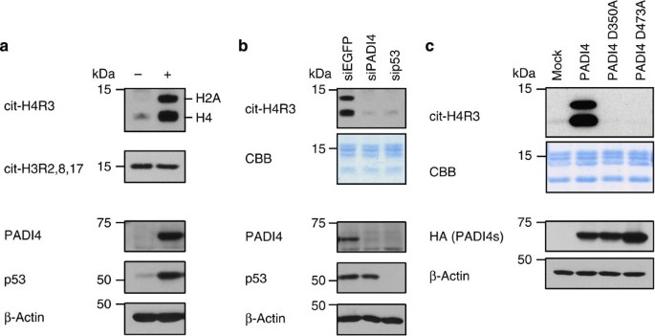Figure 2: Citrullination of histone H4R3 in the damaged cells. (a) Western blotting for histones extracted from ADR-treated U-2 OS cells (lane 2) using antibodies against citrullinated histone H4R3 (cit-H4R3) or citrullinated histone H3R2,8,17 (cit-H3R2,8,17). Whole-cell extracts were subjected to immunoblotting with anti-PADI4, anti-p53 or anti-β-actin antibody. U-2 OS cells without ADR treatment were used as a control (lane 1). (b) siRNA against PADI4 or p53 was transfected 10 h before ADR treatment. siEGFP was used as a control. Extracted histones were immunoblotted with anti-cit-H4R3 antibody. Whole-cell extracts were subjected to immunoblotting with anti-PADI4, anti-p53 or anti-β-actin antibody. CBB staining was shown to ensure equal loading. (c) Histones were extracted from HEK293T cells transfected with plasmid-expressing HA tagged-wild-type PADI4, mutant PADI4 (D350A or D473A), or mock and immunoblotted with anti-cit-H4R3 antibody. Whole-cell extracts were subjected to immunoblotting with anti-HA or anti-β-actin antibody. Figure 2: Citrullination of histone H4R3 in the damaged cells. ( a ) Western blotting for histones extracted from ADR-treated U-2 OS cells (lane 2) using antibodies against citrullinated histone H4R3 (cit-H4R3) or citrullinated histone H3R2,8,17 (cit-H3R2,8,17). Whole-cell extracts were subjected to immunoblotting with anti-PADI4, anti-p53 or anti-β-actin antibody. U-2 OS cells without ADR treatment were used as a control (lane 1). ( b ) siRNA against PADI4 or p53 was transfected 10 h before ADR treatment. siEGFP was used as a control. Extracted histones were immunoblotted with anti-cit-H4R3 antibody. Whole-cell extracts were subjected to immunoblotting with anti-PADI4, anti-p53 or anti-β-actin antibody. CBB staining was shown to ensure equal loading. ( c ) Histones were extracted from HEK293T cells transfected with plasmid-expressing HA tagged-wild-type PADI4, mutant PADI4 (D350A or D473A), or mock and immunoblotted with anti-cit-H4R3 antibody. Whole-cell extracts were subjected to immunoblotting with anti-HA or anti-β-actin antibody. Full size image We also found the citrullination of histone H3 at its N terminus in non-treated U-2 OS cells and HEK293T cells ( Supplementary Fig. S1 ), but these modifications were hardly detectable with anti-MC antibody, probably because of the low sensitivity of this antibody to the citrullination at its N terminus of histone H3 ( Fig. 1a,c ). Although citrullination of H3 was slightly increased by ectopic expression of PADI4 or by ADR treatment, siPADI4 did not affect H3-citrullination level ( Supplementary Fig. S1 ). Because citrullination of H3 was observed in HEK293T and U-2 OS cells without any stresses, we suspect that other PADI family members might also be involved in H3 citrullination in these cells. Localization of citrullinated histone H4 at fragmented nuclei To investigate the physiological role of PADI4-mediated histone citrullination, we examined chromatin structure and subcellular localization of cit-H4R3 in PADI4-introduced HEK293T cells. Immunocytochemical analysis revealed the weak and irregular staining of nuclei with 4,6-diamidino-2-phenylindole (DAPI), a characteristic feature of chromatin decondensation ( Fig. 3a ). In contrast, cit-H4R3 displayed a dot-like staining pattern around the decondensed nuclei in cells expressing HA-PADI4 ( Fig. 3a ). Fractionation of chromatin obtained from PADI4-introduced HEK293T cells [21] suggested that cit-H4R3 was enriched in S1 (soluble in divalent metal; transcriptional active) and S2 (soluble in EDTA; transcriptional inactive) fractions, compared with P fraction (insoluble compact chromatin) ( Fig. 3b ). As apoptosis is associated with dynamic changes of nuclear structure, we examined the localization cit-H4R3 in apoptotic cells. At 48 h after treatment with ADR, cit-H4R3 was localized around the fragmented nuclei in U-2 OS cells, but it was not detected in the cells, additionally treated with siRNA against PADI4 ( Fig. 3c,d ). Similar results were observed in ADR-treated MCF7 cells ( Supplementary Fig. S2a,b ). In addition, cit-H4R3 expression was significantly correlated with the level of apoptosis induction demonstrated by the TdT-mediated dUTP nick end labeling (TUNEL) assay in ADR-treated U-2 OS cells ( Fig. 3e ). These findings indicated that cit-H4R3 was associated with the decondensed soluble chromatin in apoptotic cells. 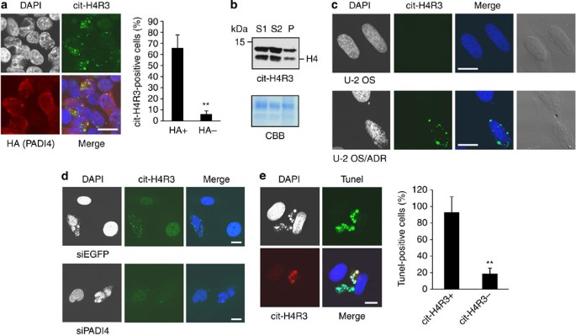Figure 3: Localization of cit-H4R3 around the fragmented nuclei during apoptosis. (a) Representative image of HA-PADI4-transfected HEK293T cells stained with anti-citrullinated histone H4R3 (cit-H4R3) antibody (Alexa Fluor 488) and anti-HA antibody (Aleza Fluor 594) (left panel).The proportion of cit-H4R3-positive cells stratified by HA-PADI4 expression was indicated (right panel). Error bars represent s.d. (n=4). **P<0.01 by Student'st-test. Scale bars, 20 μm. (b) Chromatin fractionation followed by western blotting. Isolated nuclei from HEK293T cells transfected with PADI4-expressing plasmids were digested with MNase. Digested nuclei were fractionated into three fractions: transcriptionally active (S1), transcriptionally inactive (S2) and insoluble compact chromatin (P). Aliquots from S1, S2 and P fractions were separated by SDS–PAGE and then analysed by western blotting using anti-cit-H4R3 antibody. (c) Representative image of ADR-treated U-2 OS cells stained with anti-cit-H4R3 antibody (Alexa Fluor 488). Cells were treated with 2 μg ml−1of ADR for 2 h and fixed 48 h later. Scale bars, 20 μm. (d) Representative image of ADR-treated U-2 OS cells stained with anti-citrullinated histone H4R3 antibody (Alexa Fluor 488). Each cell line was treated with 2 μg ml−1of ADR for 2 h and fixed 48 h later. Each siRNA was transfected 10 h before the ADR treatment. siEGFP was used as a control. Scale bars, 20 μm. (e) Co-staining of U-2 OS cells with TUNEL (FITC) and anti-cit-H4R3 antibody (Alexa Fluor 594) at 48 h after treatment with 2 μg ml−1of ADR for 2 h (left panel). The proportion of TUNEL positive cells stratified by cit-H4R3 expression was indicated (right panel). Error bars represent s.d. (n=7). **P<0.01 by Student'st-test. Scale bars, 20 μm. Figure 3: Localization of cit-H4R3 around the fragmented nuclei during apoptosis. ( a ) Representative image of HA-PADI4-transfected HEK293T cells stained with anti-citrullinated histone H4R3 (cit-H4R3) antibody (Alexa Fluor 488) and anti-HA antibody (Aleza Fluor 594) (left panel).The proportion of cit-H4R3-positive cells stratified by HA-PADI4 expression was indicated (right panel). Error bars represent s.d. ( n =4). ** P <0.01 by Student's t -test. Scale bars, 20 μm. ( b ) Chromatin fractionation followed by western blotting. Isolated nuclei from HEK293T cells transfected with PADI4-expressing plasmids were digested with MNase. Digested nuclei were fractionated into three fractions: transcriptionally active (S1), transcriptionally inactive (S2) and insoluble compact chromatin (P). Aliquots from S1, S2 and P fractions were separated by SDS–PAGE and then analysed by western blotting using anti-cit-H4R3 antibody. ( c ) Representative image of ADR-treated U-2 OS cells stained with anti-cit-H4R3 antibody (Alexa Fluor 488). Cells were treated with 2 μg ml −1 of ADR for 2 h and fixed 48 h later. Scale bars, 20 μm. ( d ) Representative image of ADR-treated U-2 OS cells stained with anti-citrullinated histone H4R3 antibody (Alexa Fluor 488). Each cell line was treated with 2 μg ml −1 of ADR for 2 h and fixed 48 h later. Each siRNA was transfected 10 h before the ADR treatment. siEGFP was used as a control. Scale bars, 20 μm. ( e ) Co-staining of U-2 OS cells with TUNEL (FITC) and anti-cit-H4R3 antibody (Alexa Fluor 594) at 48 h after treatment with 2 μg ml −1 of ADR for 2 h (left panel). The proportion of TUNEL positive cells stratified by cit-H4R3 expression was indicated (right panel). Error bars represent s.d. ( n =7). ** P <0.01 by Student's t -test. Scale bars, 20 μm. Full size image PADI4 promotes DNA fragmentation In neutrophils, histone hypercitrullination is known to mediate NET formation that is associated with highly decondensed chromatin structures [22] . As chromatin decondensation was shown to increase the accessibility of DNase, we hypothesized that PADI4 promotes nuclear fragmentation. Micrococcal nuclease (MNase), which can digest chromatin at the linker DNA region into solubilized poly- and mono-nucleosome-size fragments, was used to evaluate the accessibility of DNA as well as chromatin compaction. MNase treatment of purified chromatin produced fragmented-nucleosomes more effectively in cells transfected with wild-type PADI4 than those with mutant PADI4 or mock ( Fig. 4a ). This result was confirmed by SDS–PAGE in which core histones from soluble nucleosome were stained with Coomassie brilliant blue (CBB) ( Fig. 4b ). ADR treatment also enhanced DNA cleavage (evaluated by histones in soluble nucleosome), but pretreatment with the siPADI4 remarkably suppressed MNase-mediated DNA digestion ( Fig. 4c ). Taking these observations into account, our findings revealed that PADI4 increased the accessibility of DNA and subsequently promoted the DNA fragmentation. 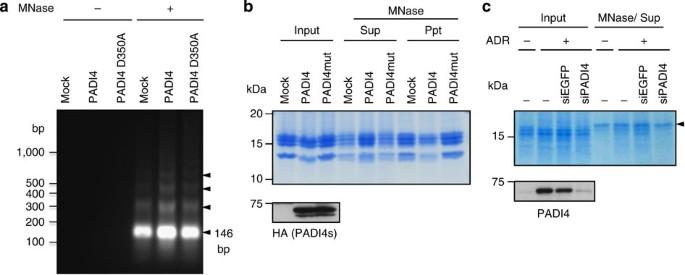Figure 4: Regulation of DNA cleavage by PADI4. (a) Chromatin was isolated from HEK293T cells transfected with PADI4 expressing plasmid. Chromatin extracted from equal numbers of cells was digested with MNase at 37 °C for 2 min. Soluble DNA released from MNase-treated chromatin were subjected to agarose gel electrophoresis. Arrow heads denote mono- and poly-nucleosomal DNAs. (b) Chromatin was isolated from HEK293T cells transfected with PADI4-expressing plasmid. Chromatin extracted from equal numbers of cells was digested with MNase at 37 °C for 2 min. Soluble core histones released from MNase-treated chromatin were subjected to SDS–PAGE. CBB staining for input chromatin is shown as controls. Input chromatin was subjected to immunoblotting with anti-HA antibody. (c) Chromatin was isolated from U-2 OS cells treated with ADR. Each siRNA was transfected 10 h before DNA damage treatment. siEGFP was used as a control. Chromatin extracted from equal numbers of cells was digested with MNase at 37 °C for 2 min. Soluble core histones released from MNase-treated chromatin were subjected to SDS–PAGE. CBB staining for input chromatin is shown as controls. Input chromatin was subjected to immunoblotting with anti-PADI4 antibody. Arrow head indicates MNase. Figure 4: Regulation of DNA cleavage by PADI4. ( a ) Chromatin was isolated from HEK293T cells transfected with PADI4 expressing plasmid. Chromatin extracted from equal numbers of cells was digested with MNase at 37 °C for 2 min. Soluble DNA released from MNase-treated chromatin were subjected to agarose gel electrophoresis. Arrow heads denote mono- and poly-nucleosomal DNAs. ( b ) Chromatin was isolated from HEK293T cells transfected with PADI4-expressing plasmid. Chromatin extracted from equal numbers of cells was digested with MNase at 37 °C for 2 min. Soluble core histones released from MNase-treated chromatin were subjected to SDS–PAGE. CBB staining for input chromatin is shown as controls. Input chromatin was subjected to immunoblotting with anti-HA antibody. ( c ) Chromatin was isolated from U-2 OS cells treated with ADR. Each siRNA was transfected 10 h before DNA damage treatment. siEGFP was used as a control. Chromatin extracted from equal numbers of cells was digested with MNase at 37 °C for 2 min. Soluble core histones released from MNase-treated chromatin were subjected to SDS–PAGE. CBB staining for input chromatin is shown as controls. Input chromatin was subjected to immunoblotting with anti-PADI4 antibody. Arrow head indicates MNase. Full size image p53–PADI4 citrullinates Lamin C at its carboxy terminus Next, we introduced PADI4 into HEK293T cells and performed immnunocytochemical analysis using anti-MC antibody. The results clearly indicated the citrullination of nuclear membrane proteins in cells expressing HA-PADI4 ( Fig. 5a ). Lamin family proteins are the main components of the nuclear lamina and are essential for various nuclear processes including apoptosis. Western blotting using nuclear extracts from PADI4-introduced HEK293T cells revealed the band shift of Lamin C protein, but not those of other Lamin proteins ( Fig. 5b ). Furthermore, we detected the citrullination of immunopurified Lamin C protein from PADI4-introduced HEK293T cells using anti-MC antibody ( Fig. 5c ). Because Lamins A and C share 566 amino acids of their N-terminal portions, six carboxy-terminal amino acids (VSGSRR) specific for Lamin C is likely to contain a target(s) of citrullination ( Supplementary Fig. S3a ). Hence, we constructed plasmids expressing various types of mutant Lamin C and examined the citrullination of each mutant protein. Western blotting with anti-MC antibody revealed that substitution of both 571st and 572nd arginine residues caused a significant reduction of protein citrullination ( Fig. 5d ). Accordingly, we raised an antibody against citrullinated Lamin C at these two arginine residues ( Supplementary Fig. S3b ). This antibody clearly recognized the citrullinated Lamin C in PADI4-introduced HEK293T cells as well as ADR-treated U-2 OS cells ( Fig. 5e ). In addition, immunocytochemistry revealed that the citrullinated Lamin C was localized predominantly around the fragmented nuclei in the damaged U-2 OS ( Fig. 5f ) and MCF7 cells ( Supplementary Fig. S4a ). Furthermore, cit-Lamin C expression was significantly correlated with the apoptotic cells in ADR-treated U-2 OS cells ( Supplementary Fig. S4b ), suggesting the involvement of citrullination of Lamin C in the nuclear fragmentation during apoptosis. 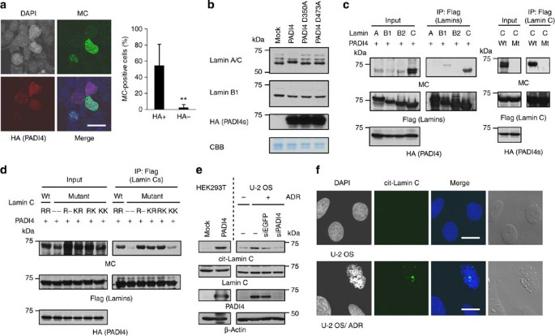Figure 5: Lamin C is citrullinated during nuclear fragmentation. (a) Representative image of HA-PADI4-transfected HEK293T cells stained with anti-modified citrulline (MC) antibody (Alexa Fluor 488) and anti-HA antibody (Aleza Fluor 594) (left panel). The proportion of MC-positive cells stratified by HA-PADI4 expression was indicated (right panel). Error bars represent s.d. (n=9). **P<0.01 by Student'st-test. Scale bars, 20 μm. Cells were incubated with 5 μmol l−1of A23187 for 1 h before fixation. (b) Western blotting for nuclear extracts from HEK293T cells transfected with wild-type PADI4, mutant PADI4 (D350A or D473A), or mock plasmid using each anti-Lamin antibody. (c) HEK293T cells were transfected with the indicated plasmids. Cell extracts were immunoprecipitated using anti-Flag antibody, followed by immunoblotting with anti-MC, anti-Flag, or anti-HA antibody. (d) HEK293T cells were transfected with the indicated plasmids. Cell extracts were immunoprecipitated using anti-Flag antibody, followed by immunoblotting with anti-MC, anti-Flag, or anti-HA antibody. (e) Whole-cell extracts from PADI4-transfected HEK293T cells or ADR-treated U-2 OS cells were subjected to western blotting using antibody against citrullinated Lamin C at arginine 571 and arginine 572 residues (cit-Lamin C), Lamin C, PADI4, or β-actin. Each siRNA was transfected 10 h before DNA damage treatment. siEGFP was used as a control. (f) Representative image of ADR-treated U-2 OS cells stained with anti-cit-Lamin C antibody (Alexa Fluor 488). Scale bars, 20 μm. Taken together, PADI4 could mediate the critical steps of apoptotic cell death through the citrullination of the core histones and Lamin C. Figure 5: Lamin C is citrullinated during nuclear fragmentation. ( a ) Representative image of HA-PADI4-transfected HEK293T cells stained with anti-modified citrulline (MC) antibody (Alexa Fluor 488) and anti-HA antibody (Aleza Fluor 594) (left panel). The proportion of MC-positive cells stratified by HA-PADI4 expression was indicated (right panel). Error bars represent s.d. ( n =9). ** P <0.01 by Student's t -test. Scale bars, 20 μm. Cells were incubated with 5 μmol l −1 of A23187 for 1 h before fixation. ( b ) Western blotting for nuclear extracts from HEK293T cells transfected with wild-type PADI4, mutant PADI4 (D350A or D473A), or mock plasmid using each anti-Lamin antibody. ( c ) HEK293T cells were transfected with the indicated plasmids. Cell extracts were immunoprecipitated using anti-Flag antibody, followed by immunoblotting with anti-MC, anti-Flag, or anti-HA antibody. ( d ) HEK293T cells were transfected with the indicated plasmids. Cell extracts were immunoprecipitated using anti-Flag antibody, followed by immunoblotting with anti-MC, anti-Flag, or anti-HA antibody. ( e ) Whole-cell extracts from PADI4-transfected HEK293T cells or ADR-treated U-2 OS cells were subjected to western blotting using antibody against citrullinated Lamin C at arginine 571 and arginine 572 residues (cit-Lamin C), Lamin C, PADI4, or β-actin. Each siRNA was transfected 10 h before DNA damage treatment. siEGFP was used as a control. ( f ) Representative image of ADR-treated U-2 OS cells stained with anti-cit-Lamin C antibody (Alexa Fluor 488). Scale bars, 20 μm. Full size image Padi4 −/− mice exhibits apoptosis resistance To further investigate the physiological function of Padi4, we generated Padi4 −/− mice ( Supplementary Fig. S5 ). Padi4 −/− mice were grossly normal in terms of survival, physical appearance and organ morphology. Then, we prepared messenger RNAs of thymuses from γ-ray-irradiated mice. The result of quantitative real-time PCR demonstrated that Padi4 mRNA was significantly increased after DNA damage in wild-type mice but not in Padi4 -deficient mice, compared with p21 Waf1 as a positive control ( Fig. 6a ). We also detected the γ-ray-induced PADI4 expression in U-2 OS cells in a dose-dependent manner ( Supplementary Fig. S6a ). Immunohistochemical analysis of in vivo citrullination of H4R3 in Padi4 +/+ mice exhibited the significant signal of cit-H4R3 in thymus at 24 h after γ-ray irradiation, although cit-H4R3 was not detected in Padi4 −/− mice ( Fig. 6b ). Concordantly, the numbers of TUNEL-positive and cleaved caspase-3-positive-cells were decreased in Padi4 −/− mice ( Fig. 6c,d ). We also found that X-ray irradiation induced expressions of mouse Padi4 and human PADI4 in a p53-dependent manner ( Supplementary Fig. S6b–d ). Subsequently, we examined by western blotting, the level of cleaved caspase-3 in X-ray-irradiated thymus and found the significant reduction of cleaved caspase-3 in Padi4 −/− mice ( Fig. 6e ), further supporting a critical role of Padi4 in the apoptotic process. 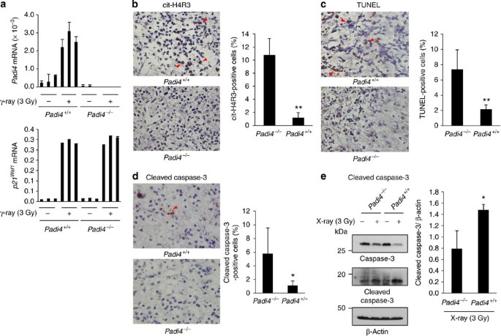Figure 6: The role of Padi4 in DNA damage induced apoptosisin vivo. (a) Quantitative real-time PCR analysis ofPadi4andp21Waf1expression in thymuses from γ-ray-irradiatedPadi4−/−orPadi4+/+mice (3 Gy). Error bars represent range (n=2).Gapdhwas used for normalization ofPadi4expression levels. Mice were sacrificed 24 h after irradiation with 3 Gy of γ-ray. (b) Representative images of thymus sections from γ-ray-irradiatedPadi4−/−orPadi4+/+mouse 24 h after irradiation with 3 Gy of γ-ray stained for citrullinated histone H4R3 (cit-H4R3) (left panel, X40). The proportion of positive cells inPadi4−/−orPadi4+/+mouse was indicated (right panel). Error bars represent s.d. (n=4). **P<0.01 by Student'st-test. (c) Representative images of TUNEL staining for thymus sections from γ-ray-irradiatedPadi4−/−orPadi4+/+mouse 24 h after irradiation with 3 Gy of γ-ray (left panel, X40). The proportion of positive cells inPadi4−/−orPadi4+/+mouse was indicated (right panel). Error bars represent s.d. (n=4). **P<0.01 by Student'st-test. (d) Representative images of cleaved-caspase-3 staining in thymus sections from γ-ray-irradiatedPadi4−/−orPadi4+/+mouse 24 h after irradiation with 3 Gy of γ-ray (left panel, X40). The proportion of positive cells inPadi4−/−orPadi4+/+mouse was indicated (right panel). Error bars represent s.d. (n=4). *P<0.05 by Student'st-test. (e) Whole-cell extracts of thymus from X-ray-irradiatedPadi4−/−orPadi4+/+mice were subjected to immunoblotting with anti-cleaved caspase-3, anti-caspase-3 or anti-β-actin antibody (left panel). Mice were sacrificed 48 h after irradiation with 3 Gy of X-ray. The ratio between cleaved caspase-3 and β-actin from independent samples (n=4 forPadi4−/−mice andn=2 forPadi4+/+mice) was indicated (right panel). *P<0.05 by Student'st-test. Figure 6: The role of Padi4 in DNA damage induced apoptosis in vivo . ( a ) Quantitative real-time PCR analysis of Padi4 and p21 Waf1 expression in thymuses from γ-ray-irradiated Padi4 −/− or Padi4 +/+ mice (3 Gy). Error bars represent range ( n =2). Gapdh was used for normalization of Padi4 expression levels. Mice were sacrificed 24 h after irradiation with 3 Gy of γ-ray. ( b ) Representative images of thymus sections from γ-ray-irradiated Padi4 −/− or Padi4 +/+ mouse 24 h after irradiation with 3 Gy of γ-ray stained for citrullinated histone H4R3 (cit-H4R3) (left panel, X40). The proportion of positive cells in Padi4 −/− or Padi4 +/+ mouse was indicated (right panel). Error bars represent s.d. ( n =4). ** P <0.01 by Student's t -test. ( c ) Representative images of TUNEL staining for thymus sections from γ-ray-irradiated Padi4 −/− or Padi4 +/+ mouse 24 h after irradiation with 3 Gy of γ-ray (left panel, X40). The proportion of positive cells in Padi4 −/− or Padi4 +/+ mouse was indicated (right panel). Error bars represent s.d. ( n =4). ** P <0.01 by Student's t -test. ( d ) Representative images of cleaved-caspase-3 staining in thymus sections from γ-ray-irradiated Padi4 −/− or Padi4 +/+ mouse 24 h after irradiation with 3 Gy of γ-ray (left panel, X40). The proportion of positive cells in Padi4 −/− or Padi4 +/+ mouse was indicated (right panel). Error bars represent s.d. ( n =4). * P <0.05 by Student's t -test. ( e ) Whole-cell extracts of thymus from X-ray-irradiated Padi4 −/− or Padi4 +/+ mice were subjected to immunoblotting with anti-cleaved caspase-3, anti-caspase-3 or anti-β-actin antibody (left panel). Mice were sacrificed 48 h after irradiation with 3 Gy of X-ray. The ratio between cleaved caspase-3 and β-actin from independent samples ( n =4 for Padi4 −/− mice and n =2 for Padi4 +/+ mice) was indicated (right panel). * P <0.05 by Student's t -test. Full size image Frequent missense mutations of PADI4 in cancer cell lines To verify the biological and clinical significance of PADI4 in human carcinogenesis, we performed DNA sequencing of the PADI4 gene in 22 breast, 21 colorectal and 37 lung cancer cell lines ( Supplementary Table S1 ). We identified six missense mutations in six cell lines, among which the wild-type PADI4 allele was lost in three cell lines ( Supplementary Fig. S7a ). As these mutations were not likely to affect the mRNA expression level ( Supplementary Fig. S7b ), we constructed plasmid vectors expressing either of six mutant PADI4 proteins and transfected either of these plasmids into HEK293T cells. Although T79 mutation did not affect enzymatic activity, five of six mutations lead to the remarkable decrease in enzymatic activity ( Fig. 7a ). Interestingly, T79 was not strictly conserved, while other five mutations were highly conserved among 14 mammalian species ( Supplementary Table S2 ). These findings suggested the complete loss of PADI4 activity in MDA-MB-435S and SK-BR-3 cells. In concordance with this result, ectopic expression of p53 using adenovirus vector expressing p53 (Ad-p53) in MDA-MB-435S cells did not induce H4R3 citrullination, while H4R3 citrullination was observed in MDA-MB-231 cells in which wild-type PADI4 was retained ( Fig. 7b ). Moreover, citrullination of H4R3 was significantly associated with apoptosis induction of Ad-p53-infected MDA-MB-231 cells ( Supplementary Fig. S7c ), indicating a critical role of PADI4-mediated histone H4 citrullination in a p53-related pathway. Similarly, Ad-p53 infection enhanced citrullination of Lamin C only in cells in which both PADI4 alleles are intact ( Supplementary Fig. S7d ). Because PADI4 was expected to function as a homodimer [23] , our findings suggested that mutant PADI4 would exhibit dominant-negative activity. Although PADI4 was mutated in LoVo cells, citrullination of Lamin C was remarkably increased in these cells. We assume that PADI1 , PADI2 and PADI3 belonging to the PADI family might mediate the citrullination of Lamin C in LoVo cells because of relatively high levels of expression of these three members ( Supplementary Fig. S7e ). 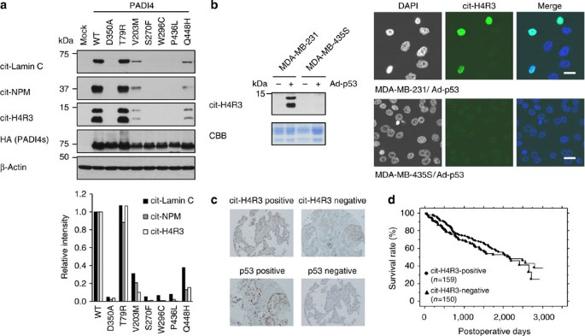Figure 7: Involvement of PADI4 in carcinogenesis. (a) Whole-cell extracts from HEK293T cells transfected with wild-type or mutant PADI4 were subjected to western blotting using anti-citrullinated Lamin C (cit-Lamin C), anti-citrullinated nucleophosmin (cit-NPM), anti-citrullinated histone H4R3 (cit-H4R3), anti-HA, or anti-β-actin antibody (upper panel). For quantification, band intensities were normalized to the signal in cells transfected with wild-type PADI4 (lower panel). (b) MDA-MB-231 and MDA-MB-435S cells were infected with adenovirus vector expressing p53 (Ad-p53). Histones were subjected to western blotting using anti-cit-H4R3 (left panel). Representative images of Ad-p53-infected cells stained for cit-H4R3 is shown in right panel. Scale bars, 20 μm. (c) cit-H4R3 or p53 expression in NSCLC tissues (magnification X10). (d) Kaplan–Meier analysis of survival in patients with NSCLC according to the expression of cit-H4R3 (P=0.24, log-rank test). Figure 7: Involvement of PADI4 in carcinogenesis. ( a ) Whole-cell extracts from HEK293T cells transfected with wild-type or mutant PADI4 were subjected to western blotting using anti-citrullinated Lamin C (cit-Lamin C), anti-citrullinated nucleophosmin (cit-NPM), anti-citrullinated histone H4R3 (cit-H4R3), anti-HA, or anti-β-actin antibody (upper panel). For quantification, band intensities were normalized to the signal in cells transfected with wild-type PADI4 (lower panel). ( b ) MDA-MB-231 and MDA-MB-435S cells were infected with adenovirus vector expressing p53 (Ad-p53). Histones were subjected to western blotting using anti-cit-H4R3 (left panel). Representative images of Ad-p53-infected cells stained for cit-H4R3 is shown in right panel. Scale bars, 20 μm. ( c ) cit-H4R3 or p53 expression in NSCLC tissues (magnification X10). ( d ) Kaplan–Meier analysis of survival in patients with NSCLC according to the expression of cit-H4R3 ( P =0.24, log-rank test). Full size image PADI4 is a potential tumour suppressor We examined the citrullination of H4R3 by tissue microarrays consisting of 309 NSCLC tissues ( Fig. 7c ). Clinicopathological analysis revealed that cit-H4R3 was associated with smaller tumour size ( P =0.0136 by Student's t -test, Table 1 ). We also found that 5-year survival rate in patients with cit-H4R3 expression (58.1%) was slightly longer than that in patients without cit-H4R3 expression (52.7%), although the difference was not statistically significant ( P =0.24 by log-rank test; Fig. 7d ). As many of p53 mutations lead to a prolonged half-life of p53 protein, immunohistochemistry of p53 is commonly used to detect p53 mutations in various cancers [24] , [25] . Interestingly, the positive p53 staining was inversely associated with cit-H4R3 staining ( P =0.0079 by Student's t -test), indicating the regulation of chromatin modification by p53 in human carcinogenesis ( Table 1 ). Table 1 Association between citrullinated H4R3-positivity and clinicopathological parameters in NSCLC patients. Full size table Accumulating evidence indicate that a combination of genetic and epigenetic alterations contribute to the development and progression of human cancers [26] . Among many genes altered in cancer tissues, the p53 gene was mutated in nearly half of all tumours [27] , [28] , [29] ; however, the roles of p53 in histone modifications and chromatin structure have not been characterized. Here we clearly demonstrated the crucial roles of p53–PADI4 pathway in citrullination of H4R3 and Lamin C in response to DNA damage as well as in nuclear fragmentation. A certain type or a combination of histone modifications termed as 'histone code' [30] are translated into a meaningful biological outcome such as gene expression and chromatin structure. Histone H2AX is phosphorylated at serine 139 residue (γ-H2AX) on external damage, and recruits DNA repair complex to promote chromatin remodelling [31] , [32] . Recently, phosphorylation of serine 14 residue in H2B, which was induced on several apoptotic stimuli including DNA damage [33] , was proposed as a 'death code, but its physiological significance remains to be determined. Histone methylation, phosphorylation and acetylation are reversible processes that are regulated by histone-modifying enzymes [34] . In contrast, citrullination is a chemically stable modification, and decitrullination enzymes have not yet been discovered [35] . Therefore, histone citrullination is considered to be an irreversible cellular process. As histone H4 citrullination is associated with apoptosis of damaged cells as well as neutrophilic death triggered by NET formation, histone H4 citrullination could be defined as a functional apoptotic histone code. Li et al . previously reported that PADI4 negatively regulated the p21 WAF1 expression through the interaction with p53 at a p21 WAF1 promoter region in ultraviolet-irradiated U-2 OS cells [36] . In addition, PADI4 was shown to be transactivated in various cancer tissues [37] , and siPADI4 or PADI4 inhibitor (Cl-amidine) suppressed proliferation of U-2 OS cells [36] , suggesting PADI4 to function as an oncogene. However, the frequent inactivating mutations of PADI4 in cancer cell lines as well as apoptosis-resistance in Padi4 -null mice implied the possible role of PADI4 as a tumour suppressor. This discrepancy could be partially due to the difference in the experimental conditions. We analysed the effects of PADI4 knockdown using irradiated mice or ADR-treated cells, whereas Li et al . analysed U-2 OS cells under the non-stress condition or after ultraviolet treatment. Although ADR- or γ-ray-treatment remarkably increased PADI4 expression, ultraviolet-treatment did not induce PADI4 expression in U-2 OS cells ( Supplementary Fig. S8a ). In addition, expression levels of p21 Waf1 in thymus in the Padi4 +/+ and Padi4 −/− mice after γ-ray irradiation were not significantly different ( Fig. 6a ). Similarly, siPADI4 treatment did not affect the expression of p53-target genes including p21 WAF1 in ADR-treated U-2 OS cells ( Supplementary Fig. S8b ). Moreover, siPADI4-treated U373MG cells exhibited resistance to p53-induced apoptosis ( Supplementary Fig. S8c ). In fact, we observed the citrullination of histone H4R3 in 51.5% of lung cancer tissues, suggesting the activation of PADI4 in a large proportion of cancer tissues, as suggested in the previous report [37] . However, cancer tissues are persistently exposed to oxidative stress compared with adjacent normal tissues [38] , [39] , activation of PADI4 would be related with cellular stress condition. Taken together, we assume that PADI4 could predominantly function as a tumour suppressor that mediates the apoptotic process of damaged cells. Although the molecular mechanism of how PADI4 increases DNA accessibility was not fully elucidated, loss of positive charge by citrullination was shown to induce conformational changes of histone H4 N terminal [40] . DNA–histone interaction is charge-dependent, and changes in the charge of the histone tails are considered to weaken histone-DNA interaction [41] . Moreover, we found that the interaction between core histones and nucleophosmin was inhibited by citrullination ( Supplementary Fig. S8d ). Any or all of these changes can affect the structure and folding of individual nucleosome that could lead to a more open and permissive chromatin environment. The role of PADI4 in chromatin remodelling was shown in the previous papers [42] , [43] . We also reported that DNA damage induced PADI4 expression and the citrullination of various proteins in our previous study [10] . To our knowledge, this is the first report demonstrating the important role of histone H4R3 citrullination in human carcinogenesis and the p53-mediated apoptotic pathway. Cell culture and transfections Cell lines were purchased from American Type Culture Collection, Lonza Biologics, or Japanese Collection of Research Bioresources. Cells were transfected with plasmids using FuGENE6 (Roche). Replication-deficient recombinant viruses Ad-p53 or Ad-LacZ, expressing p53 or LacZ, respectively, were generated and purified, as described previously [5] . siRNA oligonucleotides, commercially synthesized by Sigma Genosys, were transfected with Lipofectamine RNAiMAX reagent or Lipofectamine 2000 reagent (Invitrogen). Sequences of oligonucleotides are shown in Supplementary Table S3 . For treatment with calcium ionophore, cells were incubated with 5 μM of A23187 (Calbiochem) for 1 h at 37 °C. Plasmid construction Complementary DNA fragments of Lamin A, Lamin B1, Lamin B2 and Lamin C were amplified and cloned into pCAGGS vector. PADI4 expression plasmids were previously described [10] . Plasmids expressing mutant PADI4 or Lamin C were generated using the inverse PCR methods or by using the reverse primer containing point mutation at either or both of arginine 571 and 572 residues, respectively. The primer sequences for cloning and mutagenesis are shown in Supplementary Table S3 . Knockout mice We amplified a 5,837 bp fragment containing exon 1 and exon 2 of Padi4 using C57BL/6 genomic DNA as a template. The targeting vector was designed to replace exon 1 and 2, including the transcription initiation site, by mouse PGK-1 promoter and the neomycin-resistance gene ( Supplementary Fig. S5a ). We introduced the linearized targeting vector by electroporation into embryonic stem cells, and identified two independent targeted 129S1 embryonic stem cell clones by Southern blot analysis. We generated chimeric males by the aggregation method and crossed them with C57BL/6 females, and verified germline transmission by Southern blot analysis ( Supplementary Fig. S5b,c ). All Padi4 −/− mice used in this study had been backcrossed for ten generations into the C57BL/6 background. We used RT–PCR to determine the presence of the Padi4 transcript ( Supplementary Fig. S5d ). p53-deficient mice were provided from RIKEN BioResource Center (Ibaragi, Japan) [44] . Genotypes were confirmed by PCR analysis. The primer sequences are indicated in Supplementary Table S3 . All mice were maintained under specific pathogen-free conditions and were handled in accordance with the Guidelines for Animal Experiments of the Institute of Medical Science (University of Tokyo, Tokyo, Japan). DNA damaging treatment For treatment with genotoxic stress, cells were continuously incubated with 2 μg ml −1 ADR for 2 h, γ-irradiated using a Cs-137 source (Gamma cell-40, Atomic energy of Canada), ultraviolet-irradiated using an ultraviolet cross-linker (XL-1500, Spectronics corporation), or X-irradiated using an X-ray irradiation system (MBR-1520R-3, Hitachi). Mice were also γ-irradiated using a Cs-137 source (Gamma cell-40, Nordion) or X-irradiated using an X-ray irradiation system (MBR-1520R-3, Hitachi). Quantitative real-time PCR Peripheral blood mononuclear cells were obtained by separating blood cells in a Ficoll gradient (Amersham). Peripheral blood mononuclear cells were incubated with phytohaemagglutinin for 72 h and exposed to an X-ray irradiation. Total RNA was isolated from mouse tissue or human cells using RNeasy spin column kits (Qiagen) according to the manufacturer's instruction. Blood RNA of irradiated mice was prepared using Mouse RiboPure-Blood RNA Isolation Kit (Ambion). Complementary DNAs were synthesized with the SuperScript Preamplification System (Invitrogen). Quantitative real-time PCR was conducted using the SYBR Green I Master on a LightCycler 480 (Roche). The primer sequences are indicated in Supplementary Table S3 . Immunoprecipitation Cell extracts from HEK293T cells transfected with plasmids encoding Flag-Lamins and/or HA-PADI4s were prepared by adding HBST buffer (10 mM HEPES at pH 7.4, 150 mM NaCl and 0.5% TritonX-100). Extracts were precleared by incubation with protein G-Sepharose 4B (Zymed) and mouse IgG at 4 °C for 1 h. Precleared cell extracts were then incubated with anti-Flag affinity gel (Sigma) at 4 °C for 2 h. The beads were washed 4 times with 1 ml of ice-cold HBST buffer, and immunoprecipitated proteins were released from the beads by boiling in sample buffer for 2 min. Western blotting To prepare whole-cell extracts, cells or tissues were lysed in chilled HBST buffer for 30 min on ice and centrifuged at 16,000 g for 15 min. Histones were purified in acidic condition as previously described [45] . Samples were subjected to SDS–PAGE and immunoblotting using standard procedures. To detect citrullinated proteins, blots of deiminated proteins were treated with medium for chemical modification at 37 °C for 3 h, and, then, modified citrulline residues were detected with an anti-modified citrulline antibody (anti-MC antibody, Upstate). Bands were quantified by the Image J software. Antibodies To develop an antibody against Cit571-572 Lamin C, a Lamin C peptide (LHHHHVSGSCitCit) was chemically synthesized and used to immunize rabbits. The positive antisera were further purified by immune-affinity purification using a Lamin C Cit571-572 peptide. Anti-citrullinated nucleophosmin (NPM) antibody was prepared as previously described [10] . Polyclonal anti–MC antibody (17-347) and anti-citrullinated arginine 3 of histone H4 antibody (07-596) were purchased from Upstate. Anti-β-actin monoclonal antibody (A5441) and Anti-Flag monoclonal (F3165) and polyclonal (F7425) antibodies were purchased from Sigma. Anti-p53 monoclonal antibody (OP140) and anti-Lamin B antibody (NA12) were purchased from Calbiochem. Anti-HA monoclonal (sc-7392) and polyclonal (sc-805) antibodies were purchased from Santa Cruz Biotechnology. Anti-HA rat monoclonal antibody (3F10) was purchased from Roche. Anti-6×His monoclonal antibody (631212) was purchased from Clontech. Anti-PADI4 polyclonal antibody (ab50332), anti-citrullinated histone H3 antibody (ab5103) and anti-mono methyl histone H4 antibody (ab17339) were purchased from Abcam. Anti-Lamin A/C antibody (#2032 or #4777), anti-caspase-3 antibody (#9662) and anti-cleaved caspase-3 (#9661) were purchased from Cell signaling. List of antibodies and the concentrations used are shown in Supplementary Table S4 . In vitro citrullination assay Recombinant histone proteins were purchased from Millipore. Glutathione S -transferase (GST) fusion PADI4 and NPM1 proteins were generated as previously described [10] . His-tagged proteins were generated by cloning of their coding sequences into pET21a or pET28a vector (Novagen). Proteins were expressed in Escherichia coli and purified on Ni-NTA agarose (Qiagen) by standard methods. Deimination reactions were carried out as previously described [10] . GST pull-down assay Core histones were purified from HEK293T cells using Histone Purification Kit (Active motif). GST-NPM (1 μg) and core histones (1 μg) were separately incubated with PADI4 (1 μg) or PADI4-D350A (1 μg) for 1 h at 37 °C with 1 mM of CaCl2. PADI4-treated NPM1 and histones were mixed and stored on ice for 1 h. The mixture was incubated at 4 °C for 2 h with 20 μl of a glutathione–Sepharose 4B bead suspension (Amersham Pharmacia). After the beads were washed extensively, proteins were eluted from the beads by incubation with SDS sample buffer, separated by SDS–PAGE, and visualized by silver staining. Immunocytochemistry Immunocytochemistry was performed as previously described [10] . Before incubating with anti-MC antibody, cells were treated with medium for chemically modifying citrulline residues at 37 °C for 3 h. For co-staining of TUNEL and citrullinated proteins, cells were immunostained followed by TUNEL reaction for 1 h at 37 °C using the kit ( In Situ Cell Death Detection Kit, Fluorescein, Roche). Quantification was performed by counting around 100 cells from more than 4 independent fields. Immunohistochemistry Frozen sections of mouse thymus were used for immunohistochemistry and TUNEL staining. Immunohistochemistry was performed using the immunohistochemistry EnVision (Dako) method. TUNEL staining was performed using Apoptosis in situ Detection Kit (Wako) according to the manufacturer's instruction. Tissue microarrays were constructed in our laboratory, and staining and statistical analysis were performed as previously described [46] . Mutation analysis Genomic DNA was purified from 80 cancer cell lines by standard protocol [8] . The list of cell lines is shown in Supplementary Table S1 . 16 coding exons of the PADI4 gene were amplified, purified and sequenced. The sequences of primers used in this analysis are indicated in Supplementary Table S3 . Chromatin fractionation S1, S2 and P chromatin fractions from HEK293T cell nuclei were prepared according to previously described procedures [47] with minor modifications. HEK293T cells were transfected with PADI4-expressing plasmid. The collected cells were incubated in cell homogenization buffer (10 mM Tris at pH 8.0, 10 mM MgCl 2 , 0.5% NP40 and 1 mM DTT) on ice for 10 min. The nuclear pellet was obtained by centrifugation and resuspended in MNase digestion buffer (15 mM Tris pH 7.4, 15 mM NaCl, 60 mM KCl, 0.25 M sucrose, 1 mM CaCl 2 ). The pellet was then treated with MNase (New England Biolabs) for 2 min at 37 °C. The solution was centrifuged to obtain the supernatant (S1). The pellet was resuspended in 0.1 mM EDTA, incubated at 4 °C for 30 min, and centrifugated to obtain the chromatin fraction (P) and supernatant (S2). The proteins contained in each fraction were separated by 15% SDS–PAGE and detected by western blotting. MNase assay The nuclear pellet (Input) was treated with MNase as shown above. The reaction was terminated by adding the stop solution (0.5 mM EGTA, 25 mM EDTA). After centrifugation at 14,000 g for 5 min, DNA was extracted from the aqueous phase and analysed on agarose gel. Histone proteins collected from the aqueous phase (Sup) and pellet (Ppt) were separated by SDS–PAGE. Cell death assay Cells were infected with 20 multiplicity of infection (MOI) of Ad-p53 at 7 h after transfection of siRNA oligonucleotide. 60 h after infection cells were incubated with TUNEL reaction mixture for 1 h at 37 °C using the kit ( In Situ Cell Death Detection Kit, Fluorescein, Roche). Apoptotic cells were quantified by fluorescence-activated cell sorting analysis. How to cite this article: Tanikawa, C. et al . Regulation of histone modification and chromatin structure by the p53–PADI4 pathway. Nat. Commun. 3:676 doi: 10.1038/ncomms1676 (2012).